Magnetic order in a frustrated two-dimensional atom lattice at a semiconductor surface Two-dimensional electron systems, as exploited for device applications, can lose their conducting properties because of local Coulomb repulsion, leading to a Mott-insulating state. In triangular geometries, any concomitant antiferromagnetic spin ordering can be prevented by geometric frustration, spurring speculations about ‘melted’ phases, known as spin liquid. Here we show that for a realization of a triangular electron system by epitaxial atom adsorption on a semiconductor, such spin disorder, however, does not appear. Our study compares the electron excitation spectra obtained from theoretical simulations of the correlated electron lattice with data from high-resolution photoemission. We find that an unusual row-wise antiferromagnetic spin alignment occurs that is reflected in the photoemission spectra as characteristic ‘shadow bands’ induced by the spin pattern. The magnetic order in a frustrated lattice of otherwise non-magnetic components emerges from longer-range electron hopping between the atoms. This finding can offer new ways of controlling magnetism on surfaces. Geometric frustration and its interplay with strong electronic correlations has long been a subject of very active research, since Anderson [1] suggested that a spin-1/2 Heisenberg antiferromagnet (AF) on the triangular lattice would have a gapless quantum spin liquid ground state, that is, a resonant valence bond state. Quite generally, this interplay is believed to be the source of a variety of exotic phases in triangular systems: examples span from the possible quantum spin liquid state in κ -(ET) 2 Cu 2 (CN) 3 (refs 2 , 3 ) over to a magnetically ordered Mott insulator, which provides the parent phase for the superconductivity found in κ -(BEDT-TTF) 2 X organics [4] , [5] and Na x CoO 2 ˙ y H 2 O (ref. 6 ), with the latter having possibly a topological superconductivity phase, that is, a gap structure breaking time-reversal symmetry [7] . One key issue, which has recently been intensively studied, is the possibility of a magnetically ordered state appearing despite the frustration and, in particular, how to pin down its appearance in a convincing theoretical and experimental manner. The possibility of an ordered magnetic state in a spatially anisotropic triangular AF has received special interest for the spin-1/2 Heisenberg AF: for nearly isotropic exchange ( , where J and are the anisotropic nearest-neighbour couplings) this model displays long-range spiral order, in accordance with strong-correlation studies of the corresponding Hubbard models with isotropic hopping [8] , [9] . Several studies have proposed that, as is enhanced, that is, anisotropy introduced, quantum fluctuations destroy this order and induce an 2D spin liquid phase [9] . Therefore, it came as a substantial surprise that order, that is, a collinear AF (CAF) state, was stabilized in the spatially anisotropic AF at small , in particular, as it is unusual for quantum fluctuations to stabilize an ordered state of higher classical energy [10] . In this study, we verify that the CAF state can be achieved even in an isotropic triangular lattice from a different perspective, including additional hopping processes beyond nearest neighbours. The latter situation is obviously very relevant for realistic frustrated materials, such as the actual adatom system on a semiconductor surface, that is, Sn/Si(111)- , which we consider here. In a previous work [11] , we found that, by including the next-nearest-neighbour hopping as dictated by density functional theory (DFT) calculations, the magnetic spin susceptibility indicates an instability not towards the 120° AF, that is, spiral order, but towards the CAF state. The earlier conjecture of a CAF pattern is made here rather concrete by combining a dynamical cluster approximation (DCA) plus DFT theoretical analysis of the single-particle spectral function of the triangular lattice Sn/Si(111) system with high-precision angle-resolved photoelectron spectroscopy (ARPES). In particular, the ordered collinear magnetic structure can be identified in the ARPES spectra in terms of ‘shadow bands’ (that is, spectral weight redistributions) induced by the collinear spin pattern. This establishes the single-particle spectral function and the combination of up-to-date many-body calculations with high-precision ARPES as a powerful tool for extracting spin patterns in frustrated magnets. The adatom system Sn/Si(111)- , with its triangular lattice arrangement ( Fig. 1a ) of Sn atoms on top of Si(111), provides an ideal playground for studying geometric frustration in the presence of strong electronic correlations: a dip in the conductance at the Fermi level, which was observed in scanning tunnelling spectroscopy at low temperature [12] together with the theoretical calculations [11] , [13] , [14] , [15] reveal that indeed correlations are strong and drive the system into a Mott metal-insulator transition. 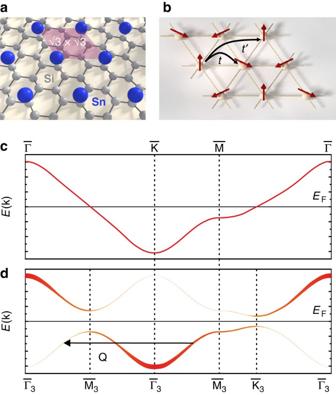Figure 1: Electron correlations in a triangular lattice. (a,b): Schematic presentation of the-Sn/Si(111) surface and the isotropic triangular antiferromagnet in the case of a spiral AF order (: electron-hopping parameters). (c) The single QP bandE(k) in the Fermi liquid regime corresponding to our LDA surface band. (d) QP (heavy line) and shadow band (light line) induced by the Mott metal-insulator transition. Figure 1: Electron correlations in a triangular lattice. ( a , b ): Schematic presentation of the -Sn/Si(111) surface and the isotropic triangular antiferromagnet in the case of a spiral AF order ( : electron-hopping parameters). ( c ) The single QP band E ( k ) in the Fermi liquid regime corresponding to our LDA surface band. ( d ) QP (heavy line) and shadow band (light line) induced by the Mott metal-insulator transition. Full size image In such a geometrically frustrated lattice arrangement, any magnetic ordering may be prevented. In this case, one may expect a spin liquid, which is a magnetic system that has ‘melted’ because of quantum fluctuations, even at zero temperature. However, in our combined theoretical and experimental work, the realization of a frustrated triangular arrangement of Sn adatoms on a Si(111) surface yields instead an ordered CAF state. The key mechanism that drives the formation of magnetic order in an otherwise non-magnetic surface are electron-hopping processes beyond nearest-neighbour atoms in the presence of strong electronic correlations. Effect of magnetic order on the electronic states Let us start out with the possibility of a magnetically ordered 120° AF (that is, spiral) state, as indicated in Fig. 1 , and its influence on the quasi-particle (QP) spectral function A ( k , E ). This spiral magnetic reconstruction pattern corresponds to a (3 × 3) reconstruction ( Fig. 1b ), while the CAF order, after the three rotations (see Fig. 3b) preserving the lattice symmetry (domain averaging), results in a reconstruction. In the Fermi liquid regime, which may be here taken as our surface band from the local density approximation (LDA) (see below) crossing the Fermi energy E F , the QP peak of A ( k , E ) defines a single energy E ( k ) for each value of k in the first surface Brillouin zone (SBZ), as shown in Fig. 1c . When a spin-density wave (SDW) is present, as in Fig. 1d , k is mixed with k + Q by exchange Bragg scattering, where Q is the magnetic ordering vector. This creates energy eigenstates | Ψ k , which no longer have a sharp momentum, that is, | Ψ k = u k | k + v k | k + Q , with , where | k , | k + Q are the (for example, LDA) eigenstates of Fig. 1c , u k , v k denote the standard coherence factors of BCS theory, which describe here the SDW gap features introduced by AF order [16] . The energy spectrum of the | Ψ k states is schematically drawn in Fig. 1d , where the states denoted by a heavy line carry a large weight, that is, , and the states denoted by a light line carry the small weight . Thus, if one creates a hole of energy E ( k ) in the lower band by ARPES, one will observe the emitted electron having momenta k with probability and ( k + Q ) with probability . Hence, the SDW Bragg scattering leads to a shadow band, displaced by Q in Fig. 1d , a celebrated phenomenon observed for example, for the high- T c cuprates in the square-lattice AF, that is, undoped situation [16] . Many-body modelling of strong electron correlations We now turn to the Sn/Si(111) surface system. Before we discuss our results in Figs 2 , 3 , 4 , a few remarks are in order about our theoretical and experimental set-ups, both of which are more detailed in the Methods section and in the Supplementary Information , that is, Supplementary Figs S1–S4 . 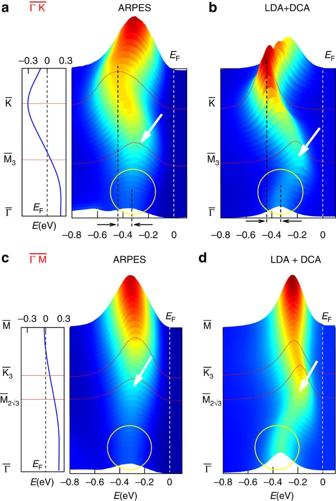Figure 2: Spectral function from photoemission and many-body theory. Comparison of the ARPES data (T≈60 K,hv=130 eV) in (a,c) with the spectral functions from LDA+DCA calculations in (b,d), alonganddirections, respectively. White arrows indicate band maxima, which are not present in the metallic LDA-derived bands (see LDA plots, left-hand side), but are created by the Mott-insulating state, characterized by shadow bands. Yellow circles aroundhighlight these shadow bands observed in both ARPES and in the LDA+DCA calculations. Figure 2: Spectral function from photoemission and many-body theory. Comparison of the ARPES data ( T ≈60 K, hv =130 eV) in ( a , c ) with the spectral functions from LDA+DCA calculations in ( b , d ), along and directions, respectively. White arrows indicate band maxima, which are not present in the metallic LDA-derived bands (see LDA plots, left-hand side), but are created by the Mott-insulating state, characterized by shadow bands. Yellow circles around highlight these shadow bands observed in both ARPES and in the LDA+DCA calculations. 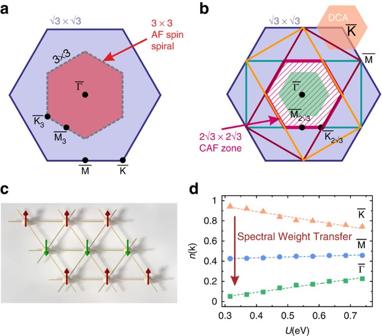Figure 3: Collinear antiferromagnetic ordering. (a,b) Magnetic-order induced zone boundaries for the-Sn/Si(111) SBZ, (a) with 120° AF, (b) with CAF order in three-fold rotational superposition, leading to an effectiveSBZ. (c) Row-wise spin alignment of the CAF order. (d) Spectral weight transfer (see arrow) consistent with shadow bands induced by the CAF superstructure. Full size image Figure 3: Collinear antiferromagnetic ordering. ( a , b ) Magnetic-order induced zone boundaries for the -Sn/Si(111) SBZ, ( a ) with 120° AF, ( b ) with CAF order in three-fold rotational superposition, leading to an effective SBZ. ( c ) Row-wise spin alignment of the CAF order. ( d ) Spectral weight transfer (see arrow) consistent with shadow bands induced by the CAF superstructure. 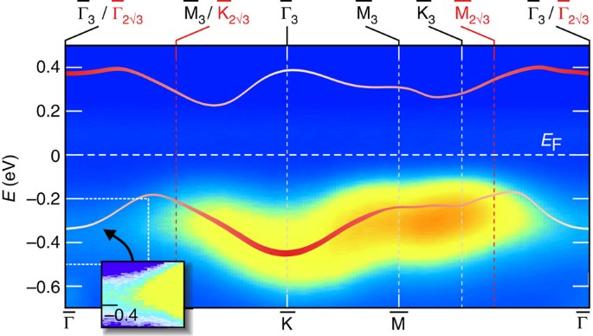Figure 4: Band back-folding in magnetically ordered state. Comparison of the (LDA+DCA) QP dispersion (red curve) with the ARPES intensity (false colour plot) in the originalSBZ (lower labels) and the (3 × 3) andSBZs (upper labels). Inset: replica of the ARPES shadow band within dashed box, displayed with enhanced contrast, which highlights the non-degeneracy betweenand. Full size image Figure 4: Band back-folding in magnetically ordered state. Comparison of the (LDA+DCA) QP dispersion (red curve) with the ARPES intensity (false colour plot) in the original SBZ (lower labels) and the (3 × 3) and SBZs (upper labels). Inset: replica of the ARPES shadow band within dashed box, displayed with enhanced contrast, which highlights the non-degeneracy between and . Full size image In our theoretical description, we start from a DFT (LDA) electronic structure calculation of a slab configuration of (six) Si-layers, with the Sn atoms placed on the top-layer in equivalent ( T 4 ) lattice positions. This is in agreement with geometrical structure determinations using X-ray diffraction [17] . In particular, it excludes any additional lattice superstructure, for example, a (3 × 3) lattice periodicity. For technical reasons (see Methods) the Si bottom-layer is saturated by H-atoms. In the next step, the Sn-related surface band (shown in Fig. 1c ) is projected onto a maximally localized Wannier function (MLWF) basis from which the dominant electronic hopping parameters t and as indicated in Fig. 1b are derived and a single-band Hubbard model is constructed [11] . This model is then solved employing the DCA [18] , with the continuous-time quantum Monte Carlo method [19] as a ‘cluster solver’. Details of the (LDA+DCA) methodology can again be found in the Methods section. Finally, to determine the strength of the electronic correlations, the corresponding Coulomb interaction U ~0.66 eV was chosen so as to achieve best agreement for the local density of states (DOS) between theory and experiment ( Supplementary Fig. S4 ). Using this U -value, our approach starts from the gapped correlated state. The spin-susceptibility calculations [11] suggest a magnetic, that is, collinear order. Here, we perform a detailed study of the single-particle excitation, which, in terms of the shadow bands and their spectral weight transfer ( Figs 2 , 3 ), provides firm support for the collinear state. Experimentally, the Sn/Si(111) system, with a surface reconstruction of high quality as verified by low-energy electron diffraction (LEED) and scanning tunnelling microscopy (STM), was exposed to ARPES carried out at the Advanced Light Source in Berkeley. The photoelectrons were detected with an energy resolution of 25 meV throughout all measurements (see Methods section). Spectral function with shadow bands Figure 2 summarizes our main findings for both the experimental (ARPES) and theoretical (LDA+DCA) k -resolved photoemission spectra along two high-symmetry directions (that is, and ). A rather good overall agreement emerges from this comparison, on the basis of which we can confidently extract the existence of an unexpected new magnetic order, that is, the CAF order: (i) The upper row ( Fig. 2a ) for seems first to convey the existence of a (3 × 3) reconstruction pattern in accordance with the 120° AF order of Fig. 1b and the SDW-derived bands displaying both large and small spectral weights, as schematically depicted in Fig. 1d . In particular, we find the shadow bands between the and -symmetry points of the (3 × 3) SBZ (depicted in Fig. 3a ) carrying the characteristically small spectral weights. These shadow band regions are observed in both ARPES and in the (LDA+DCA) calculations. They are highlighted close to the point by the four yellow circles in Fig. 2 . This is contrasted by the LDA bands, which are in this k -space regime above the Fermi energy, not contributing to the photoemission spectral weight. Closer inspection reveals another structure just below −0.6 eV close to the -point, which is a bulk band of the Si(111) substrate (see Li et al . [11] ) and not a surface band and, therefore, not relevant to the surface magnetic pattern. So, at a first glance, the appearance of the shadow band seems to modify the spectral dispersion from to a (3 × 3) symmetry, which could, in principle, be consistent with a spiral SDW ( Fig. 1b ) or a (3 × 3) surface reconstruction [20] , [21] . (ii) However, closer inspection of Fig. 2 reveals a more complex and exciting underlying reconstruction pattern: first of all, if a (3 × 3) symmetry would be realized, then a ‘smoking-gun’ test would be that the energy value of the shadow band at the -point should be degenerate, that is, at the same energy as the QP band at the -point. This is clearly not the case in Fig. 2a , both in experiment and in theory (see black vertical dashed lines). Thus, within the theoretical calculation and, independently, within the ARPES data, we observe about a tenth of an eV energy ‘offset’ between - and -points. On the scale of the bandwidth of ~0.3 eV, this is a relevant energy difference and, therefore, allows us to identify the magnetic structure from the electron band symmetries. (iii) The white arrows in Fig. 2 indicate the new SDW-induced band maxima not present in the LDA-derived bands. The maxima appear at the transition point from a large to a small spectral weight (for example, around the -symmetry point in Fig. 2a ). Further support that the (3 × 3) symmetry is not realized comes from the observation (more pronounced in the theoretical results in Fig. 2d ) that, along the symmetry direction , the transition point (white arrow) is not located in the close vicinity of the (3 × 3) symmetry point , but at a new symmetry point, denoted by in Fig. 2c . In summary, both ARPES experiment and theory rule out a (3 × 3) reconstruction, which could be of the spiral 120° AF magnetic origin as illustrated in Fig. 1b . Similarly, a (3 × 3) lattice reconstruction, which has also been discussed for the Sn/Si(111) adatom system [20] , [21] , is excluded by both our LDA+DCA calculation where all Sn atoms are located at equivalent lattice sites, and the non-degeneracy (in Fig. 2 ) of the bands at and positions. Redistribution of spectral weight and magnetic order Next, we provide a second part of our ‘smoking-gun’ test, which concerns our Mott–Hubbard physical picture, that is, that a magnetic order appears in the strongly correlated Sn/Si(111) system despite the obvious lattice frustration. This is illustrated in Fig. 3 where the effective surface SBZs for 120° AF (excluded) and CAF orders [11] are depicted in panels (a) and (b), respectively. Figure 3c illustrates the row-wise spin alignment in real space. A characteristic fingerprint is the formation of shadow bands and the related spectral shifts, for example, the spectral weight shift from the momentum region around the -point to the region around the -point (just as in Fig. 1c ). Such an analysis can straightforwardly be performed in our LDA+DCA scheme by extracting the average occupation number n ( k ) at each momentum sector, that is, . As before, A ( k , E ) denotes the spectral function in the sector around k and f ( E , T ) the Fermi function, thus, n ( k ) is a measure of the spectral weight below E F in a momentum sector defined by the vector k . n ( k ) is plotted in Fig. 3d as a function of the correlation strength U for three different momentum-space areas termed , and , as indicated in Fig. 3b for the examples of the small hexagons around the - and -points. The three momentum sectors arise naturally from the underlying lattice symmetry in our 9-site DCA scheme (see Supplementary Fig. S3 ). This scheme is based on ‘coarse graining’ the k -space (here the SBZ), into 9 sections. The technical details of this procedure are not essential and, thus, are relegated to the Methods section. Very importantly, the inclusion of next nearest-neighbour hoppings in the presence of electron correlations inherently leads to AF ordering, where strong interactions are found to favour CAF order [11] . What is of relevance here is that we observe an increase of (around the point) with increasing interaction U , while (around the point) behaves exactly the opposite. In contrast, stays almost constant. This is exactly what one expects in a Mott–Hubbard type of metal-insulator transition, driven by strong correlations. The momentum region around the -point transfers spectral weight to the -point region (see Fig. 1c ), thereby creating the lower Hubbard band now visible as a shadow band in photoemission below E F . The constant demonstrates even further that this spectral weight transfer occurs between - and -regions. This part of our test, thus, proves the existence of correlation (SDW)-induced shadow bands and concomitant spectral weight transfer. To discriminate between the (3 × 3)-type spiral AF order and CAF order with effective symmetry, we refer to the first part of our analysis based on Fig. 2 , which clearly argues for the latter case. To make this point even more transparent, we overlay in Fig. 4 the ARPES intensity (false colour plot) with our theoretical (LDA+DCA) QP peak dispersion (red colour). Again, we can read off the good overall agreement and we find that the shadow band at the point is not degenerate, that is, at the same energy, as the QP band at the point. This degeneracy would only happen if the band would be back-folded by the (3 × 3) magnetic order of Fig. 1b , that is, the spiral (120°) AF order. Again, this part of the analysis clearly rules out (3 × 3) order. On the other hand, back-folding, according to the collinear SBZ in Fig. 3b , results in agreement between theory and experiment. Taken together with our earlier conjecture for a CAF (that is, the row-wise AF), based on spin-susceptibility calculations [11] , this indeed establishes the collinear magnetic order in an isotropic triangular AF. We note, that a CAF order has recently been detected also in the triangular lattice AF CuFeO 2 (ref. 22 ), in which a collinear 4-sublattice AF order is realized in 2D-planes, however, embedded in a 3D-environment. In summary, this work demonstrates that a comparison of high-precision ARPES with state-of-the-art theoretical calculations, which combine first-principle electronic structure (LDA) with cluster many-body (DCA) calculations, allows for detailed insight and determination of complex spin patterns in frustrated magnetic systems. This has been demonstrated here for the model system Sn/Si(111), which can accurately be tuned by external parameters (for example, temperature T ) into a Mott metal-insulator transition with unexpected CAF order. But the key role established here for the single-particle spectral function of Sn/Si(111) goes way beyond this specific adatom surface system, and should offer a firm basis for identifying other recently much-discussed complex spin patterns in frustrated systems, and also resolve whether or not a spin liquid is stabilized by geometrical frustration. Sample preparation and ARPES experiment The Sn/Si(111)- triangular surface system, examined by ARPES, has been prepared as follows: N-type Si substrates ( ρ <0.01 Ωcm) were flashed for several times at ≈1,250 °C until a sharp (7 × 7) pattern was observed in LEED. Subsequently, 1/3 of a monolayer of tin was deposited on the substrates by electron beam evaporation from a pyrolytic boron nitride crucible. After an additional anneal at ≈700 °C the Sn/Si(111)- surface reconstruction was verified in high quality by LEED, see Supplementary Fig. S1(a) . The STM image of occupied states at room temperature ( Supplementary Fig. S1(b) ) serves as a proof of the low-defect density at the atomic scale. Sn atoms appear as bright protrusions in a hexagonal arrangement of periodicity. Importantly, we have not found any signature of a (3 × 3) or any other kind of superstructure within a large temperature range, that is, T =20–300 K, by means of LEED. This is consistent with earlier findings by STM, where the absence of a structural change down to T =6 K was stated [23] . ARPES experiments were carried out at the electronic structure factory endstation of beamline 7.01 at the Advanced Light Source, which provides helium cooling down to 10 K and is equipped with a 6-axis goniometer. Photoelectrons, excited by linearly polarized radiation, were detected with a Scienta R 4000 spherical analyser with energy resolution set as 25 meV throughout all measurements. Dynamical cluster approximation (DCA) To study the competing low-T phases in the Sn/Si(111) system, we combine an LDA Hamiltonian represented by H LDA , with an on-site Coulomb interaction, represented by a Hubbard-U term. The essential idea then is to include long-ranged hoppings (as shown in Fig. 1b of main text) and to demonstrate that they are responsible for the unexpected magnetic order. We thus start from where is the Hamiltonian of the low-energy effective band for the Sn/Si(111) surface calculated from the LDA to the DFT. ε k is well separated from the other bands and mainly due to Sn 5 p z -orbitals. This band is projected onto MLWF following the standard recipes [24] , [25] . The single-particle hopping parameters t i are then determined from the MLWF matrix elements of the Kohn–Sham (LDA) Hamiltonian, giving rise to the following dispersion relation: where t 1 =−52.7 meV. Using t 1 as the energy unit, the longer-range hoppings, which is t 2 / t 1 , t 3 / t 1 , t 4 / t 1 , t 5 / t 1 , are derived as −0.3881, 0.1444, −0.0228, −0.0318, respectively. As shown in Supplementary Fig. S2(b) , the non-interacting DOS of the tight-binding Hamiltonian equation (2) is asymmetric with respect to the Fermi level, in particular exhibiting a large intensity at the upper band edge. This is quite different from the DOS of the triangular model with only nearest-neighbour hopping. As discussed in our main text, the inclusion of the realistic higher-order hopping processes is decisive for the appearance of the CAF [11] . Equation (1) was solved by using the DCA [26] , which recovers the infinite lattice by proliferating N c -site clusters with periodic boundary condition. In DCA, to restore translational invariance within the cluster, the intercluster hopping amplitudes are modulated by the superlattice momentum as well as the intracluster hopping integrals. Supplementary Fig. S3 illustrates the first SBZ of a triangular lattice, which is dispatched into N c =9 equal-area sectors. Each red dot represents the origin of a momentum sector. An arbitrary momentum k in the original first SBZ can be expressed as a sum of the superlattice momentum and cluster momentum K , that is, . In the DCA, the Green’s function is coarse-grained [18] over the superlattice momentum , that is, The DCA self-consistency loop is closed by the Dyson equation, . To calculate the cluster self-energy from G σ ( K , iω n ) an N c -site cluster problem has to be solved. In this study, we employ the continuous-time quantum Monte Carlo method with the paramagnetic condition, that is, . It is important to note that although we consider only a 9-site cluster in our calculation, all different hopping processes in equation (2) are included in equation (3), after proliferating the 9-site cluster to infinite size in DCA. Thus, our single-band model with the longer-ranged hoppings dictated by a priori LDA calculations is different from any study of the triangular model with only the nearest-neighbour hopping. The value of the Coulomb interaction U was fixed so as to achieve the best agreement of the DOS in both the LDA+DCA and the experiment. As shown in Supplementary Fig. S4 , at U ~0.66 eV (which is slightly above U c ≈0.60 eV required for the metal-insulator transition in this system [11] , [14] ), we find a rather good agreement at all temperatures studied. According to our calculations the spectral weight at the Fermi level E F is gradually enhanced with the increase of temperature. The respective on-set temperature T c ~120 K is higher than what has been experimentally found by other groups [12] . How to cite this article: Li, G. et al . Magnetic order in a frustrated two-dimensional atom lattice at a semiconductor surface. Nat. Commun. 4:1620 doi: 10.1038/ncomms2617 (2013).